Non-hysteretic colossal magnetoelectricity in a collinear antiferromagnet The manipulation of magnetic ordering with applied electric fields is of pressing interest for new magnetoelectric devices and information storage applications. Recently, such magnetoelectric control was realized in multiferroics. However, their magnetoelectric switching is often accompanied by significant hysteresis, resulting from a large barrier, separating different ferroic states. Hysteresis prevents robust switching, unless the applied field overcomes a certain value (coercive field). Here we address the role of a switching barrier on magnetoelectric control, and identify a material, collinear antiferromagnetic and pyroelectric Ni 3 TeO 6 , in which magnetoelectric switching occurs without hysteresis. The barrier between two magnetic states in the vicinity of a spin–flop transition is almost flat, and thus small changes in external electric/magnetic fields allow to switch the ferroic state through an intermediate state in a continuous manner, resulting in a colossal magnetoelectric response. This colossal magnetoelectric effect resembles the large piezoelectric effect at the morphotropic phase boundary in ferroelectrics. For the last decade, concentrated research on multiferroics, where magnetic and ferroelectric orders coexist, has been motivated by a desire to understand the mechanisms of magnetoelectric (ME) effects [1] , [2] , [3] , [4] , [5] and to find materials with large ME effects, suitable for practical applications [6] , [7] , [8] , [9] , [10] , [11] , [12] , [13] , [14] . A very productive strategy for achieving large ME responses [15] , [16] is to benefit from a small energy difference between competing phases in the vicinity of a phase transition, where a small external stimulus may be sufficient to favour the desired phase. Utilizing the collective nature of a phase transition and this breaking of the delicate balance near a phase boundary may give rise to a large ME response to small perturbations, even if the ME coupling is intrinsically small. The large ME response can result in switching of polarization ( P ) with external magnetic fields ( H ) or magnetization ( M ) with external electric fields ( E ) (refs 6 , 9 , 10 , 17 , 18 , 19 , 20 , 21 ). In most multiferroics known to date, a large energy barrier separates different ferroic states. In this case, switching, which occurs through nucleation of new-phase domains and their expansion through domain-wall motion, is accompanied by significant hysteresis and a large coercive field needed for switching. Whereas in memory applications hysteresis allows for non-volatility, in devices such as ME sensors and oscillators hysteresis is responsible for loss and gives rise to detrimental side effects such as low precision, drift and asymmetric oscillation. To achieve a large ME effect without any significant hysteresis, here we attempt to engineer the free-energy barrier between free-energy minima corresponding to the competing states, which determine the energy of domain walls between competing-phase domains. Finding and engineering a multiferroic with an energy barrier of desirable shape (discussed in the following) open a path to optimized ME switching. Herein, we report that utilizing a collective phase transition with a desired energy barrier results in non-hysteretic colossal magnetoelectricity. Control of magnetic states by external electric fields is the type of ME effects that is relevant to real technological applications, since applying electric fields, rather than magnetic fields, is more practical in small devices. In a number of multiferroics such as R MnO 3 (ref. 22 ), BiFeO 3 (ref. 23 ), R Mn 2 O 5 (ref. 24 ) and Ca 3 CoMnO 6 (ref. 25 ), external magnetic fields can induce spin reorientation transitions that are accompanied by large changes of polarization. However, in most of these materials, magnetism is little influenced by external electric fields. Indeed, considering the ME coupling in the free energy density , the effective magnetic field induced through the application of an electric field is =−α E , and for it to match the coercive field ( H cv ), we need to apply E cv = H cv /α, which gets prohibitively large at small ME coupling α. Thus, both large ME coupling and a particular barrier shape are crucial for robust ME control. Here we experimentally demonstrate the control of magnetization by electric fields and magnetic control of polarization across the spin–flop transition in Ni 3 TeO 6 without hysteresis and discuss a model, showing that the spin–flop transition in Ni 3 TeO 6 is associated with the required switching barrier. Ni 3 TeO 6 belongs to the M 3 TeO 6 family ( M =Mn, Cu, Co, Ni) with corundum (Al 2 O 3 ) structure [26] , [27] , in which M and Te ions replace Al. Mn 3 TeO 6 shows complex incommensurate spin ordering [28] , and magnetically induced improper ferroelectricity has recently been reported in Co 3 TeO 6 (refs 29 , 30 ). Owing to its complex magnetic phase diagram, the origin of the electric polarization in Co 3 TeO 6 is still under debate. Ni 3 TeO 6 exhibits a relatively simple magnetic structure with collinear antiferromagnetic (AFM) ordering along the c axis below T N =52 K (refs 31 , 32 , 33 ). Ni 3 TeO 6 crystallizes in a polar R 3 structure with 10 atoms in a rhombohedral unit cell. As shown in Fig. 1a , layers with Ni ii 2+ O 6 /Ni iii 2+ O 6 octahedra and those with Ni i 2+ O 6 /Te 6+ O 6 octahedra alternate along the c axis. Similar to the behaviour in Ca 3 Co 2−x Mn x O 6 (ref. 34 ), the collinear up-up-down-down spin configuration is observed in the Ni i 2+ -Ni ii 2+ -N i 2+ -Ni ii 2+ network along the c axis. Ni iii 2+ spins order in parallel with Ni ii 2+ spins in the same layer. No significant ME effect was observed in a previous magnetic and dielectric study [31] . 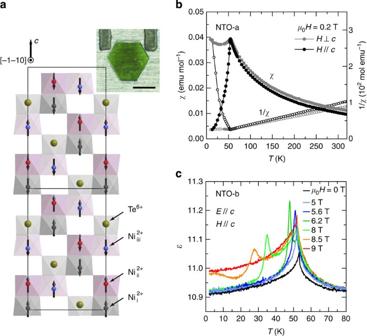Figure 1: Collinear antiferromagnetic spin structure and dielectric anomalies in Ni3TeO6. (a) Crystallographic and magnetic structures of antiferromagnetically ordered Ni3TeO6. Inset: As-grown ~100-μm-thick Ni3TeO6single crystal. Scale bar=0.5 mm. (b) Temperature dependence of DC magnetic susceptibilityχ(T) and 1/χ(T) parallel (black) and perpendicular (grey) to thecaxis of NTO-a atμH=0.2 T. (c) Temperature dependence of dielectric constant ɛ(T) of NTO-b along thecaxis at various magnetic fields applied along thecaxis. Figure 1: Collinear antiferromagnetic spin structure and dielectric anomalies in Ni 3 TeO 6 . ( a ) Crystallographic and magnetic structures of antiferromagnetically ordered Ni 3 TeO 6 . Inset: As-grown ~100-μm-thick Ni 3 TeO 6 single crystal. Scale bar=0.5 mm. ( b ) Temperature dependence of DC magnetic susceptibility χ ( T ) and 1 /χ ( T ) parallel (black) and perpendicular (grey) to the c axis of NTO-a at μ H =0.2 T. ( c ) Temperature dependence of dielectric constant ɛ( T ) of NTO-b along the c axis at various magnetic fields applied along the c axis. Full size image Here we experimentally demonstrate a non-hysteretic colossal ME (CME) control of magnetization and polarization in Ni 3 TeO 6 . In the vicinity of a spin–flop transition, an almost flat barrier between two magnetic states allows small changes in external electric or magnetic fields to switch the ferroic state through an intermediate state without hysteresis. Our Landau-type theory explains that quartic anisotropy plays an important role in the non-hysteretic ME response as well as the continuous spin–flop transition. Magnetic ordering-induced polarization The temperature dependence of the DC magnetic susceptibility parallel (χ c ) and perpendicular (χ ab ) to the c axis was measured in μ 0 H =0.2 T after zero-field cooling, as shown in Fig. 1b . Upon cooling from 320 K, both χ c ( T ) and χ ab ( T ) follow the Curie–Weiss law. At the onset temperature of the Neel transition, T N ≈55 K, χ c starts to drop and approaches zero at the zero temperature. On the contrary, χ ab exhibits a weak temperature dependence below T N . Although the observed T N ≈55 K is slightly higher than the reported T N =52 K (refs 31 , 32 , 33 ), the temperature dependence of magnetic properties is consistent with collinear AFM ordering of Ni spins along the c axis, in accordance with the result of the previous neutron-diffraction study [31] . Surprisingly, we discovered a clear dielectric anomaly at T N , evident in the temperature dependence of dielectric constant ɛ( T ) ( Fig. 1c ). In magnetic fields along the c axis up to 5.6 T, the dielectric anomaly remains intact except a slight down shift of the peak temperature. However, above μ 0 H =5.6 T, a second peak at T N′ appears. This new peak rapidly shifts to lower temperatures with increasing magnetic field, and in μ 0 H =9 T it is no longer observed. These results indicate that there exist two different magnetic states associated with different dielectric properties, and applying magnetic fields induces a transition between these ME states. Ni 3 TeO 6 is polar, and we found that the polarization of Ni 3 TeO 6 suddenly changes at magnetic transitions, as shown in Fig. 2a,b . The temperature dependence of the pyroelectric current J ( T ) in Fig. 2a shows a sharp peak feature at T N . In the case of μ 0 H =8.5 T, a broad second peak is also observed at T N′ . These J ( T ) features are consistent with the features in ɛ( T ). The induced polarization at the low temperature limit, obtained by integrating J ( T ) from T N to 2 K, is P AFM =3,280 μC m −2 ( Fig. 2b ). Considering only the Ni i 2+ -Ni ii 2+ -N i 2+ -Ni ii 2+ network, the inversion centre of the network and that of the magnetic up-up-down-down lattice do not match, and this mismatch can induce magnetic-order-induced polarization through symmetric exchange coupling. This situation resembles what happens in multiferroic Ca 3 CoMnO 6 . In μ 0 H =8.5 T, P AFM at T N′ < T < T N is slightly reduced from the zero- H (or μ 0 H =1 T) value, but P AFM is restored to the zero- H value below T N′ . P AFM in μ 0 H =9 T keeps the reduced value in the entire temperature range. Thus, the high- H state, compared with the zero- or low- H state, accompanies a reduced polarization. 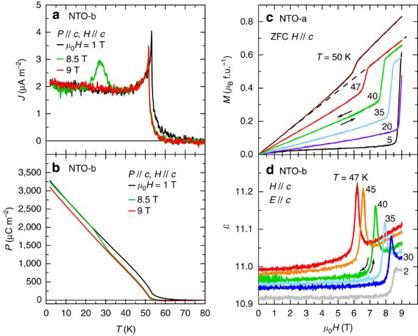Figure 2: Induced electric polarization associated with antiferromagnetism and non-hysteretic spin–flop transition. (a,b) Temperature dependence of pyroelectric currentJ(T), and electric polarizationP(T) of NTO-b determined from the integration ofJ(T) with respect to time atμH=1, 8.5 and 9 T, respectively. (c,d) Magnetic field dependence of magnetizationM(H) and dielectric constantɛ(H) of NTO-a at various temperatures for both increasing and decreasing magnetic fields. A black dashed line incdepicts linear fit toM(H) curve forH>Hcand atT=47 K. Figure 2: Induced electric polarization associated with antiferromagnetism and non-hysteretic spin–flop transition. ( a , b ) Temperature dependence of pyroelectric current J ( T ), and electric polarization P ( T ) of NTO-b determined from the integration of J ( T ) with respect to time at μ H =1, 8.5 and 9 T, respectively. ( c , d ) Magnetic field dependence of magnetization M ( H ) and dielectric constant ɛ ( H ) of NTO-a at various temperatures for both increasing and decreasing magnetic fields. A black dashed line in c depicts linear fit to M ( H ) curve for H > H c and at T =47 K. Full size image Non-hysteretic ME effect Figure 2c represents the isothermal magnetization M ( H ) along the c axis for both increasing and decreasing magnetic fields. Each M ( H ) curve shows two linear regimes and a step-like sudden increase between them at a critical magnetic field ( H c ). Upon decreasing temperature, H c increases gradually, but below 15 K it decreases slightly. M ( H ) for H > H c as well as H<H c extrapolates to zero for H =0. In addition, M ( H>H c ) /H =0.031 emu mol −1 at 47 K is comparable to χ ab ( T= 47 K)=0.038 emu mol −1 in μ 0 H =0.2 T. These observations indicate that the H -induced transition is of spin–flop-type, rather than metamagnetic. In other words, the H -induced transition accompanies a roughly 90° flop of spins, so flopped spins lie mostly in the ab plane, and the high- H state is also AFM. It indicates an archetypical spin–flop transition in an Ising antiferromagnet. However, in contrast to the spin–flop transitions in many other materials [22] , [35] , no hysteresis behaviour is observed in Ni 3 TeO 6 within our experimental accuracy. When M ( H ) is measured through varying H in a step mode, the hysteresis H at H c is less than 10 Oe even at 2 K ( Supplementary Fig. 1 ). The magnetic-field dependence of ɛ across the spin–flop transition, measured by ramping up and down in a sweep mode at various temperatures, is shown in Fig. 2d . Upon decreasing temperature, the peak of the magnetodielectric anomaly monotonically shifts to higher fields. At T =47 K the critical field in M ( H ) is μ 0 H c =6.7 T, slightly different from μ 0 H c =6.2 T in M ( H ). The slightly different critical field in ɛ( H ) and M ( H ) may stem from the strain built up during polishing of NTO-b, which is another as-grown crystal used for the ɛ( H ) measurements ( Supplementary Fig. 2b,c ). Note that even in ɛ( H ), we do not observe any magnetic field hysteresis within our experimental accuracy (<300 Oe at 2 K). Figure 4a demonstrates that P along the c axis is controlled with an external magnetic field along the c axis. 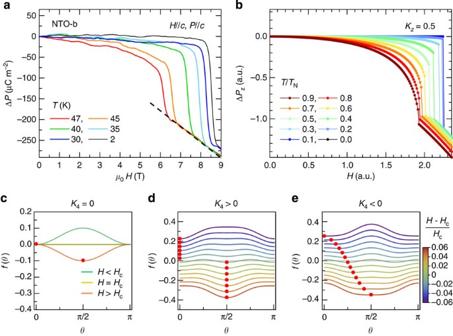Figure 4: Experimental result and calculation of magnetic field induced polarization, and magnetic field dependence of free energy. (a,b) Experimental results and theoretical calculations for the magnetic field dependence of the electric polarization ΔP(H) at various temperatures, respectively. A black dashed line inaindicates linear fit to ΔP(H) curve forH>Hcand atT=47 K. (c–e) The dependencef(θ) of the free-energy density on the direction of the antiferromagnetic order parameter for different values of fourth-order anisotropy constantK4in various magnetic fields. Free-energy minima are indicated by red dots. ForK4=0 the barrier is absent and the switching occurs instantaneously in the bulk. ForK4>0 there is a finite barrier and the transition should be of the first order with a hysteresis. IfK4<0 the minimum of the free energy shifts continuously fromθ=0 toθ=π/2 as the magnetic field increases. This case is consistent with our experimental observations. The ME effect below H c is very small, in accordance with the small longitudinal susceptibility of a collinear antiferromagnet. At the spin–flop transition P increases suddenly, and in H > H c P ( H ) exhibits a linear ME effect with a coefficient of −60 ps m −1 , consistent with a large transverse susceptibility of a collinear antiferromagnet. As shown in Fig. 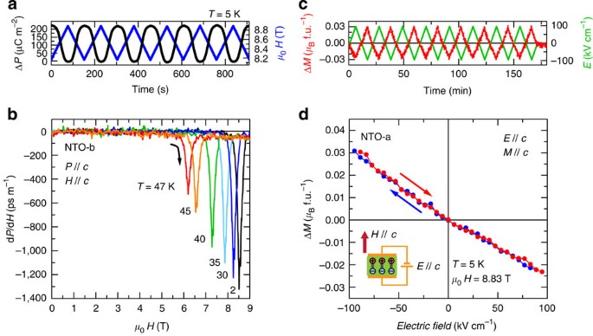3b , the ME coefficient defined by the H -derivative of P approaches −1,300 ps m −1 at H c and 2 K, and the change of P across H c is ~290 μC m −2 . Figure 3: Electric field controlled magnetization and magnetic field controlled polarization at the intermediate state. (a) Modulated electric polarization (black) as a function of time with respect to linearly varying magnetic field (blue colour) between 8.16 and 8.85 T along thecaxis at 5 K. (b) Magnetoelectric coupling constant dP/dHestimated from magnetic field derivative ofP(H) at various temperatures. (c) Modulated magnetization (red colour) along thecaxis with respect to linearly varying electric field (green colour) between +100 and −100 kV cm−1with time atT=5 K andμH=8.83 T. The electric field is applied along thecaxis. (d) Modulated magnetization, averaged over eight periods of linearly varying electric field, as a function of electric field atT=5 K andμH=8.83 T; inset illustrates the directions of applied magnetic field, electric field and polarization. Figure 3a depicts the repeated variation of P induced by a modulated magnetic field varying between μ 0 H c =8.16 and 8.85 T. At 5 K, Δ P of 225 μC m −2 oscillates with the variation of μ 0 Δ H c =0.69 T. Furthermore, the magnetization varies with a modulated electric field as demonstrated in Fig. 3c for a linearly modulated electric field between +100 and −100 kV cm −1 along the c axis. After ME cooling from 70 to 5 K with +100 kV cm −1 and 1 T, the electric field was set to zero, but the magnetic field was fixed at 8.83 T, which is H c at 5 K. Afterwards, in the presence of a modulated electric field, the magnetization oscillates linearly with the variation of 0.055 μ B f.u. −1 . Note that there exists a 180° phase shift between the external electric field and the measured magnetization. In other words, with increasing (decreasing) electric field, the magnetization decreases (increases). This is consistent with the fact that the low- H state exhibits a larger P . An averaged M ( E ) curve, obtained from repeated variation of M with a modulated electric field with eight periods, is presented in Fig. 3d , showing that the magnetization is almost linearly controlled by an electric field without hysteresis. The estimated ME coefficient of this Δ M ( E ) curve is μ 0 Δ M /Δ E =−316 ps m −1 . Figure 4: Experimental result and calculation of magnetic field induced polarization, and magnetic field dependence of free energy. ( a , b ) Experimental results and theoretical calculations for the magnetic field dependence of the electric polarization Δ P ( H ) at various temperatures, respectively. A black dashed line in a indicates linear fit to Δ P ( H ) curve for H > H c and at T =47 K. ( c – e ) The dependence f ( θ ) of the free-energy density on the direction of the antiferromagnetic order parameter for different values of fourth-order anisotropy constant K 4 in various magnetic fields. Free-energy minima are indicated by red dots. For K 4 =0 the barrier is absent and the switching occurs instantaneously in the bulk. For K 4 >0 there is a finite barrier and the transition should be of the first order with a hysteresis. If K 4 <0 the minimum of the free energy shifts continuously from θ =0 to θ = π /2 as the magnetic field increases. This case is consistent with our experimental observations. Full size image Figure 3: Electric field controlled magnetization and magnetic field controlled polarization at the intermediate state. ( a ) Modulated electric polarization (black) as a function of time with respect to linearly varying magnetic field (blue colour) between 8.16 and 8.85 T along the c axis at 5 K. ( b ) Magnetoelectric coupling constant d P /d H estimated from magnetic field derivative of P ( H ) at various temperatures. ( c ) Modulated magnetization (red colour) along the c axis with respect to linearly varying electric field (green colour) between +100 and −100 kV cm −1 with time at T =5 K and μ H =8.83 T. The electric field is applied along the c axis. ( d ) Modulated magnetization, averaged over eight periods of linearly varying electric field, as a function of electric field at T =5 K and μ H =8.83 T; inset illustrates the directions of applied magnetic field, electric field and polarization. Full size image A few other multiferroics (for example, TbMn 2 O 5 (ref. 24 ), hexaferrites [10] and (Gd,Dy,Tb)FeO 3 (ref. 9 and so on) exhibit CME effects, but those CME effects are accompanied by significant hysteresis, which is associated with first-order phase transitions. However, our experimental results demonstrate a completely different non-hysteretic CME effect associated with a continuous second-order phase transition. We emphasize that non-hysteretic ME effects are essential for numerous practical applications such as ME sensors and oscillators because any hysteresis gives rise to detrimental side effects such as high loss, low precision, drift and asymmetric oscillations. Note that a continuous modulation of magnetization with oscillating electric fields has been observed in soft magnet (Cu,Ni)B 2 O 4 (ref. 36 ). Compared with those of (Cu,Ni)B 2 O 4 (refs 36 , 37 ), the ME responses of polarization and magnetization in Ni 3 TeO 6 are ~46 and two times larger, respectively. In the following section, the mechanism of the non-hysteretic CME effect is explained by Landau free-energy analysis. This ME effect can be explained within a Landau free-energy description. The exchange striction between Ni i 2+ and Ni ii 2+ , for example, makes the Ni i 2+ -Ni ii 2+ bond length dependent on the scalar product of spins, which rapidly changes across the spin–flop transition. Since these ions are in inequivalent environments with different rigidities, and their charges may be slightly different, they induce different dipole moments, which result in a change of polarization as the magnetic state changes in an applied magnetic field (here and denote the magnetizations of antiferromagnet Ni sublattices). In fact, the calculated change of polarization ( Fig. 4b ) captures the main features of the experimentally observed polarization change ( Fig. 4a ). In the free-energy density, the symmetry-allowed coupling between sublattice magnetizations and the electric polarization has the form , with spins i and j on different antiferromagnet sublattices. This expression is invariant under global spin rotations, and thus describes exchange striction, associated with the dependence of Heisenberg exchange constant on the structural (in this case, polar) mode amplitude. Since the angle between and changes across the spin–flop transition, the exchange striction gives rise to a significant polarization change. As discussed earlier, our experimental results demonstrate the magnetic-field control of polarization. Since one of the phases separated by the spin–flop transition has considerably larger polarization than the other, the electric field can be used to favour this phase in the vicinity of the transition. We emphasize that this control of the competing phases with an electric field will be less if a significant hysteresis is involved in the transition. In order to understand this negligible hysteresis at the spin–flop transition, we illustrate the essential physics by invoking a simplified Landau-type theory. For each of the three non-equivalent Ni n 2+ ions (where n runs over the three Ni sublattices) in a 10-atom rhombohedral unit cell, we introduce the AFM order parameters , where the second index labels Ni n 2+ ions inside the magnetic unit cell, and the denotes sublattice magnetizations. Since the AFM exchange between the Ni spins is generally larger than any other energy scales such as magnetic or electric field, these three AFM order parameters rotate together across the spin–flop transition so that their mutual orientations do not change. This allows to introduce the total staggered magnetization , which we use to develop the Landau theory [38] . We model the uniform part of the Landau free-energy density by including all the symmetry-allowed terms up to fourth order in , The first term with τ = α ( T – T c ) represents a Mexican hat-shaped potential below the transition. The terms with K z and K 4 describe easy hexagonal c axis anisotropy and quartic anisotropy, and the terms with H describe the most general coupling to the external magnetic field. Microscopically, the anisotropy terms result from the spin-orbit coupling and are generally of the order and , where the spin-orbit coupling constant λ is usually much smaller than the crystal field splitting Δ cf . The total magnetization can be calculated as . We first consider the case of zero quartic anisotropy, . When a magnetic field applied along the c axis exceeds , the AFM order parameter rotates perpendicular to the easy axis in order to gain the Zeeman energy of spin canting along the field, as modelled by the term with β in Equation (1). Here θ is the angle between and the c axis. The dependence of the free energy on the direction of L is given by a sum of terms with K z and β , , shown in Fig. 4c . Importantly, at H = H c the free energy is independent of the direction; therefore, there exists no barrier for switching within the model considered here. The barrier may, however, appear due to the quartic K 4 term. Figure 4d,e ( K 4 ≠0) shows the deformation of f ( θ ) due to the K 4 term. For K 4 >0 as in Fig. 4d , as H increases the local minimum appears at θ=π /2 and shifts to lower energies, resulting in a first-order phase transition. On the other hand, in the case that K 4 <0 ( Fig. 4e ), the minimum of f ( θ ) at θ =0 turns into a Mexican hat resulting in a second-order phase transition controlled by the value of H , (the ab plane component of is the order parameter for this transition) and the free-energy minimum continuously moves from θ =0 to θ = π /2, guiding the rotation of through the transition ( Supplementary Fig. 3 ). At the second-phase transition, corresponding to the disappearance of L z , the symmetry does not change, so this transition is rather a crossover. Our experimental observations regarding M ( H ) and ɛ ( H ) are consistent with K 4 <0 scenario, where rotates continuously in the intermediate phase, analogous to the monoclinic phase at a morphotropic phase boundary (MPB) in ferroelectrics [39] . The H -derivative of M ( H ) reveals that two boundaries exist in the vicinity of the spin–flop transition down to 5 K ( Supplementary Fig. 1c ). Just as the piezoelectric response is enhanced at the MPB, here a ‘magnetic MPB’ facilitates the control of competing phases with electric/magnetic fields without hysteresis. Note that earlier direct-space imaging experiments [40] also point to the possibility of a spin–flop transition without domain-wall motion in La 1.4 Sr 1.6 Mn 2 O 7 . The absence of a barrier in this case leads to a non-hysteretic spin–flop transition. In other antiferromagnets, an intermediate state mediating two second-order spin–flop phase transitions was experimentally observed [41] , [42] , [43] , and spin–flop transitions have been investigated based on the Landau theory with many higher-order terms [38] , [44] . In addition, the CME effect resembles the colossal magnetoresistance effect in the sense that a large physical response to an external stimulus is associated with the tuning of a collective phase transition with an external stimulus. In our CME, the fourth-order magnetic anisotropy, which controls whether or not there exists the energy barrier for a spin–flop transition, plays the key role. In the case of colossal magnetoresistance, the small energy barrier (or a broad distribution of the energy barrier height) appears also relevant but may be associated with the presence of significant disorder. In conclusion, the magnetic exchange striction in Ni 3 TeO 6 results in a change of electric polarization at the onset of the AFM ordering. We found that in the presence of c direction magnetic fields, the spin–flop is initiated at a second-order phase transition and proceeds through a narrow intermediate state, similar to a monoclinic phase at the MPB, giving rise to colossal responses in ferroelectrics. The intermediate spin state in Ni 3 TeO 6 results in a non-hysteretic CME effect. Furthermore, the magnetization is linearly controlled by an electric field without hysteresis in the intermediate state of a spin–flop transition. In terms of utilizing an intermediate state for continuous magnetic modulations in electric fields, our experimental result resembles that of (Cu,Ni)B 2 O 4 (ref. 36 ). Our Landau-type theory explains that the quartic anisotropy in the vicinity of the spin–flop transition leads to non-hysteretic CME control of magnetization as well as polarization. These findings on the single-phase material may open a new path to the realization of practical ME devices with high tunability and good retention. Single crystal preparation and structure analysis Ni 3 TeO 6 single crystals were grown using a chemical vapour transport method at 700 °C for 4 days, followed by furnace cooling [31] . They are transparent hexagonal plates with green colour (~1 × 1 × 0.4 mm 3 ) as shown in the inset of Fig. 1a . Powder X-ray diffraction measurement and refinement were performed on crushed powders of a Ni 3 TeO 6 single crystal ( Supplementary Fig. 2a and Supplementary Table 1 ). a - and c - lattice constants are 5.107 and 13.762 Å, respectively. The R profile and goodness of fit for the refinement are 6.298 and 1.31, respectively. NTO-a is an as-grown Ni 3 TeO 6 single crystal, and another as-grown crystal (NTO-b) was polished down to 40 μm thickness along the c axis. Measurements All magnetic properties were measured on NTO-a. The temperature dependence of magnetization was measured in a Quantum Design MPMS-XL7. The measurements of dielectric constant (ɛ) and electric polarization ( P ) were performed on NTO-b using Quantum Design PPMS-9. ɛ was measured with oscillating electric fields applied along the c axis using a Quadtech 7600 LCR meter at 44 kHz. The temperature ( T ) (magnetic field ( H )) dependence of P was obtained by integrating pyroelectric ( J ( T )) (ME, J ( H )) current with respect to time. ME poling for J ( T ) and J ( H ) measurements was performed with E pole =50 kV cm −1 and μ 0 H =1 T. The temperature (magnetic field) dependences of ɛ and J ( T ) ( J ( H )) were measured at the 2 K min −1 warming rate (ramping magnetic field with 50 Oe s −1 ). The electric field ( M ( E )) and magnetic field ( M ( H )) dependence of magnetization were measured in the DC excitation mode of the AC magnetic susceptibility option in PPMS-9. The electric field for M ( E ) measurements was applied using a Keithley 6517B electrometer. How to cite this article: Oh, Y. S. et al . Non-hysteretic colossal magnetoelectricity in a collinear antiferromagnet. Nat. Commun. 5:3201 doi: 10.1038/ncomms4201 (2014).